Predicting sites of ADAR editing in double-stranded RNA ADAR (adenosine deaminase that acts on RNA) editing enzymes target coding and noncoding double-stranded RNA (dsRNA) and are essential for neuronal function. Early studies showed that ADARs preferentially target adenosines with certain 5′ and 3′ neighbours. Here we use current Sanger sequencing protocols to perform a more accurate and quantitative analysis. We quantified editing sites in an ∼ 800-bp dsRNA after reaction with human ADAR1 or ADAR2, or their catalytic domains alone. These large data sets revealed that neighbour preferences are mostly dictated by the catalytic domain, but ADAR2's dsRNA-binding motifs contribute to 3′ neighbour preferences. For all proteins, the 5′ nearest neighbour was most influential, but adjacent bases also affected editing site choice. We developed algorithms to predict editing sites in dsRNA of any sequence, and provide a web-based application. The predictive power of the algorithm on fully base-paired dsRNA, compared with biological substrates containing mismatches, bulges and loops, elucidates structural contributions to editing specificity. Adenosine deaminases that act on RNAs (ADARs) convert adenosines to inosines (A-to-I) in double-stranded regions of viral RNAs, and cellular pre-mRNAs and noncoding RNAs [1] , [2] , [3] . There are thousands of A-to-I editing sites in the human transcriptome [4] , in coding and noncoding regions of mRNAs [5] . When ADARs target codons they can profoundly affect the proteome. For example, 24 isoforms are possible through varying combinations of editing in 5-HT 2C serotonin receptor pre-mRNA [6] , [7] . Aberrant editing is linked to depression and suicide [8] , [9] , cancer [10] , and further, ADARs can modulate double-stranded RNA (dsRNA)-mediated gene silencing pathways [11] , [12] , [13] . Amino (N)-terminal regions of ADARs contain dsRNA-binding motifs (dsRBMs), whereas carboxy (C) termini contain a conserved catalytic domain. A crystal structure of the catalytic domain of human ADAR2 (hADAR2) has been solved [14] , as has the nuclear magnetic resonance solution structure of the two dsRBMs of rat ADAR2, in the presence or absence of dsRNA [15] , [16] . ADARs target dsRNA of any sequence, but have preferences for certain neighbouring nucleotides. Analyses of Xenopus laevis ADAR1 show a 5′ nearest neighbour preference (U=A>C>G), with no obvious 3′ nearest neighbour preference [17] . hADAR1 has been reported to show the same preferences, and hADAR2 a similar but distinct 5′ nearest neighbour preference (U≈A>C=G), as well as a 3′ nearest neighbour preference (U=G>C=A) [18] . These data have guided evaluation of editing in endogenous RNAs for years, yet were determined with techniques that allowed only a qualitative determination. In addition to preferences for neighbouring nucleotides, ADARs exhibit selectivity, whereby the number of adenosines edited in a dsRNA is affected by dsRNA length and whether base-pairing is interrupted by mismatches, bulges or loops [19] . Editing of an AU base pair (bp) creates an IU mismatch, and selectivity is thought to relate to how many mismatches a dsRNA can tolerate before becoming too single stranded to be recognized by an ADAR. In all, 50–60% of adenosines in dsRNAs longer than ∼ 50 bp can be edited before the reaction stops, whereas shorter dsRNAs are edited more selectively, at fewer sites. Internal loops can uncouple helices to turn a long dsRNA into a series of short dsRNAs that are edited more selectively [20] . Current paradigms hold that dsRBMs mediate selectivity [21] . Here we use optimized methodology to refine and quantify neighbour preferences of human ADAR1 and ADAR2. Further, by evaluating neighbour preferences of truncated proteins, we determine contributions of the catalytic domain separately from dsRBMs. Using data from in vitro editing of a long perfectly base-paired dsRNA, we develop algorithms for predicting editing sites and provide a web-based programme ( http://www.biochem.utah.edu/bass/inosinepredict ). Using this algorithm we evaluate the importance of bases beyond nearest neighbours and contributions of RNA structure. Quantification by peak height is relatively accurate DNA sequencing data are often reported in Applied Biosystems trace files ('.abi' chromatograms). Traces from cDNAs of ADAR-edited RNA have been considered to be unquantifiable [22] , as earlier dye terminator chemistry resulted in non-uniform peak heights. Advances in chemistry have improved peak-height uniformity [23] , but there has been no evaluation of newer outputs to determine adequacy for quantifying editing. To this end, we mixed PCR products representing unedited or edited sequence at known ratios to create a mixture with a defined percentage of edited sequences (see Methods ). The mixture was sequenced and chromatograms were quantified by measuring T and C peak heights in strands opposing the edited strand because A/G mixed peaks have more inconsistent heights [23] . 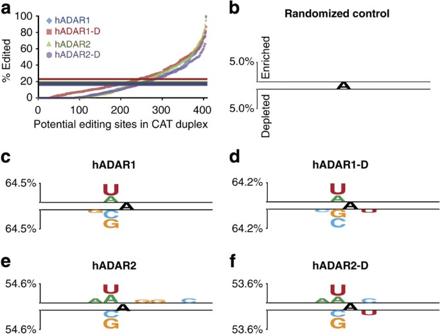Figure 1: Binary analysis using Two Sample Logo software. (a) Bulk sequencing of the 795-bp dsRNA RT–PCR product allowed measurement of 406 adenosines on the sense and antisense strands combined. The plot arranges each site in order of increasing percentage of editing measured within the population of RT–PCR products. Coloured horizontal lines show mean overall A-to-I conversion of the 795-bp dsRNA incubated with each ADAR: hADAR1 (blue)=17.8%, hADAR1-D (red)=22.7%, hADAR2 (green)=19.1% and hADAR2-D (purple)=16.4%. For Two Sample Logo analyses (b–f), sequence contexts edited to a greater extent than the mean were scored as enriched, and those edited less than the mean as depleted. Neighbour preferences of the different ADARs were determined from a single incubation, but repeated experiments showed the same relative pattern of editing among the 406 adenosines, even when protein concentrations differed between experiments. (b–f) Logo displays enriched bases above top line and depleted bases below bottom line for neighbouring five bases on both sides of the central edited adenosine. Level of enrichment/depletion is shown by letter heights with reference to scale on the left;y-axes as in (b). Two Sample Logo settings:t-test, show base ifPvalue <0.005 and no Bonferroni correction25. Panels show: (b) Two Sample Logo of Randomized Control; (c) hADAR1; (d) hADAR1-D; (e) hADAR2; and (f) hADAR2-D. The percent of the population edited at each site evaluated in the chromatogram was compared with the known ratio of unedited to edited sequences, or 'true % editing', in the prepared mixture ( Table 1 ). The least accurate measurements for the 15 sites were those for the true 60% edited mixture, which on average was low by 8% (average 52.3±4.5); measuring peak heights rather than volumes gave the least variability (see Supplementary Table S1 ). The coefficient of variation (ratio of standard deviation to mean) increased at lower % editing ( Table 1 ), and here our methodology did not distinguish between large relative differences that corresponded to small absolute differences (for example, we cannot reliably distinguish the twofold relative difference between 1 and 2% editing). Regardless, the nuclease mapping method previously used to determine ADAR preferences has a standard deviation of 12%, and the more qualitative primer extension method has up to 25% inaccuracy in % editing predicted for each site [17] , [18] . Thus, the more uniform peak heights associated with current four-dye trace chemistry allowed measurements that were more accurate and precise than previous techniques. Table 1 True versus measured editing. Full size table ADAR nearest neighbour preferences Having established that measurements of peak-heights improved accuracy and precision, we used the methodology to analyse neighbour preferences of hADAR1 and hADAR2. We also investigated the contribution of dsRBMs to neighbour preferences, using truncated proteins consisting only of the catalytic domain (hADAR1-D and hADAR2-D). Titrations were performed to determine the ADAR concentration that gave ∼ 20% overall A-to-I conversion for an internally radiolabelled, 795-bp dsRNA, in 1 h at 30 °C. With this % editing, few sites were edited to 100% in the population, ensuring that information was not lost due to saturation. These concentrations were then used in the ADAR preference assay (see Methods ), in which non-radiolabelled 795-bp dsRNA was incubated with an ADAR, RNA products purified, and reverse transcribed and amplified with the PCR. PCR products were sequenced, and traces evaluated to determine the percentage of each adenosine edited in the population. These data were used to evaluate neighbour preferences using a binary or quantitative approach. Binary approach Four-dye sequence traces of cDNA derived from ADAR products have previously been evaluated qualitatively to provide a binary scale of editing within an RNA population. That is, based on a chosen cutoff, sites are scored as unedited or edited [24] . To compare our data to such studies, adenosines in the 795-bp dsRNA were scored as edited or unedited, with the cutoff defined as the mean overall editing within the cDNA population ( Fig. 1a , horizontal lines). Figure 1: Binary analysis using Two Sample Logo software. ( a ) Bulk sequencing of the 795-bp dsRNA RT–PCR product allowed measurement of 406 adenosines on the sense and antisense strands combined. The plot arranges each site in order of increasing percentage of editing measured within the population of RT–PCR products. Coloured horizontal lines show mean overall A-to-I conversion of the 795-bp dsRNA incubated with each ADAR: hADAR1 (blue)=17.8%, hADAR1-D (red)=22.7%, hADAR2 (green)=19.1% and hADAR2-D (purple)=16.4%. For Two Sample Logo analyses ( b – f ), sequence contexts edited to a greater extent than the mean were scored as enriched, and those edited less than the mean as depleted. Neighbour preferences of the different ADARs were determined from a single incubation, but repeated experiments showed the same relative pattern of editing among the 406 adenosines, even when protein concentrations differed between experiments. ( b – f ) Logo displays enriched bases above top line and depleted bases below bottom line for neighbouring five bases on both sides of the central edited adenosine. Level of enrichment/depletion is shown by letter heights with reference to scale on the left; y -axes as in ( b ). Two Sample Logo settings: t -test, show base if P value <0.005 and no Bonferroni correction [25] . Panels show: ( b ) Two Sample Logo of Randomized Control; ( c ) hADAR1; ( d ) hADAR1-D; ( e ) hADAR2; and ( f ) hADAR2-D. Full size image Two Sample Logo sequence motifs [25] representing neighbour preferences are shown for each protein ( Fig. 1c–f ). We observed no statistically significant bias in a randomized positive and negative set of all adenosine contexts in 795-bp dsRNA ( Fig. 1b ), indicating that observed preferences were not artifacts of dsRNA sequence. Even with the less precise binary approach it is clear that, for both hADAR1 and hADAR2, the 5′ nearest neighbour has the most influence on whether an adenosine will be edited ( Fig. 1c,e ). This agrees with previous studies using other methods [17] , [18] . Also in agreement is the overlapping 5′ nearest neighbour preferences of the two enzymes, with U and A being preferred, and C and G being less preferred [18] . The catalytic-domain-only proteins showed almost identical 5′ nearest neighbour preferences as the full-length proteins ( Fig. 1d,f ). However, the binary method revealed minor differences on the 3′ side for both full-length proteins compared with their catalytic domains, and at the second neighbouring base on the 5′-side for full-length hADAR1 compared with its catalytic domain. As the binary approach sacrifices magnitude information, we sought a more quantitative approach that might reveal subtle differences. Quantitative approach Sixteen sequence contexts exist based on 5′ and 3′ nearest neighbours, and we first normalized the data (see Methods ), and plotted preferences for the 16 'triplets' using peak heights ( Fig. 2 ). Triplets for all comparisons were arranged left to right on the x axis according to hADAR1 preferences (bottom panels), and differences in % editing plotted separately (top panels). 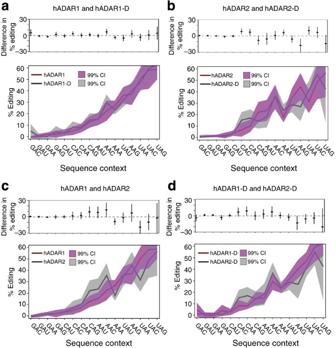Figure 2: Quantitative comparison of editing for different triplets. Bottom plots ofa–dshow the 16 possible triplet contexts on thexaxis with edited A in the centre, ordered according to hADAR1 preferences. 406 adenosines were used to determine the average percentage of the population edited in each triplet context, which is plotted on theyaxis and normalized as described (seeMethods). The 99% confidence interval (CI) for sample averages is indicated by shading. Top plots show differences in average percentage editing between compared proteins, with values for each triplet shown as black ovals and 99% confidence intervals as vertical lines. Panels show comparisons of triplet preferences for (a) hADAR1 compared with hADAR1-D, (b) hADAR2 compared with hADAR2-D, (c) hADAR1 compared with hADAR2 and (d) hADAR1-D compared with hADAR1-D. See Methods for a description of statistical methodology. Figure 2: Quantitative comparison of editing for different triplets. Bottom plots of a – d show the 16 possible triplet contexts on the x axis with edited A in the centre, ordered according to hADAR1 preferences. 406 adenosines were used to determine the average percentage of the population edited in each triplet context, which is plotted on the y axis and normalized as described (see Methods ). The 99% confidence interval (CI) for sample averages is indicated by shading. Top plots show differences in average percentage editing between compared proteins, with values for each triplet shown as black ovals and 99% confidence intervals as vertical lines. Panels show comparisons of triplet preferences for ( a ) hADAR1 compared with hADAR1-D, ( b ) hADAR2 compared with hADAR2-D, ( c ) hADAR1 compared with hADAR2 and ( d ) hADAR1-D compared with hADAR1-D. See Methods for a description of statistical methodology. Full size image All proteins showed similar trends, and a comparison of triplets along the x axis revealed a clustering of triplets according to identity of the 5′ nearest neighbour. This indicates that the 5′ nearest neighbour has the greatest influence on preferences, confirming conclusions made in our binary analysis ( Fig. 1 ) and in previous reports [17] , [18] . Triplet preferences were almost identical for hADAR1 and hADAR1-D, and very similar between hADAR2 and hADAR2-D, indicating nearest neighbour preferences are largely determined by the catalytic domain. However, hADAR2 showed a greater preference for triplets containing a 3′ G compared with its catalytic domain, hADAR2-D ( Fig. 2b ), particularly evident in analyses of CAG, AAG and UAG triplets. Thus, although the catalytic domain largely dictates nearest neighbour preferences, for hADAR2, the dsRBMs have a role in discriminating adenosines with a 3′ G. Triplet comparisons for hADAR1 and hADAR2 ( Fig. 2c ), and hADAR1-D and hADAR2-D ( Fig. 2d ), revealed that differences between the catalytic-domain-only proteins do not track with differences between the full-length proteins. This suggests that although dsRBMs do not contribute substantially to nearest neighbour preferences, the contributions differ for the two ADARs, even on perfectly base-paired dsRNA. Best-fit multiplicative models Our quantitative analysis provided data for 406 editing sites, an order of magnitude greater than used in previous analyses [17] , [18] . Using our larger data set, we set out to create models that more accurately represent neighbour preferences (see Methods ). To evaluate the predictive accuracy of various models, Table 2 shows the adjusted coefficient of determination, or R 2 , values, which estimate the percent variation in editing percentage predicted by each of six different models across the 406 editing sites. Table 2 Comparison of models for predicting neighbour preferences. Full size table Model #1, the triplet model, considered interdependent effects of 5′ and 3′ nearest neighbours, and R 2 values indicated it accounted for between 45.3% (hADAR2) and 66.5% (hADAR1-D) of the editing percentages observed for the four proteins. These R 2 values were only slightly increased compared with those for the regression fit model that considers only the 5′ nearest neighbour ( Table 2 , Model #2) reiterating that this position is most influential. Similarly, the higher R 2 values associated with hADAR1 and hADAR1-D triplet models compared with those for hADAR2 and hADAR2-D imply that hADAR1's preferences are more influenced by immediate neighbours. We next generated a best-fit model that separately takes into account the identity of 5′ and 3′ nearest neighbouring bases. The model is a two-term 7-coefficient multiplicative model that gives as accurate an R 2 value for data fit as does the triplet model with 16 coefficients ( Table 2 , compare Model #1 and #3). This model achieves greater parsimony than the triplet model by assuming that the effect of the neighbouring 5′ base does not change depending on the identity of the 3′ base, and conversely, that the effect of the neighbouring 3′ base does not change depending on the identity of the 5′ base. The similarity of the predictive power of the two-term multiplicative model to the triplet model suggests that amino acids within ADAR that interact with the 5′ side of the targeted adenosine are separate and distinct from those that interact with the 3′-side. The two-term 7-coefficient model has the form: (coefficients in Supplementary Data 1 ; see Methods ). The coefficient of 20 was used to simplify interpretation of results, in accordance with normalization of the mean % editing to 20% (see Methods ). For each ADAR, the first 3′ U coefficient was set to 1 in the regression model. The remaining three 3′ nearest neighbour coefficients, and all four 5′ nearest neighbour coefficients, were adjusted to the scale set by the 3′ U coefficient. The magnitude of coefficients in this two-term model, and associated P values for the significance of the differences between coefficients for different base identities, provide a more quantitative understanding of ADAR neighbour preferences. For example, representing these preferences in a more familiar way, the coefficients of the two-term model ( Supplementary Data 1 ) indicate that hADAR1 has the following preferences: 5′ U>A>C>G and 3′ G>C≈A>U, where the difference between 3′ C and A was not statistically significant at P ≤0.05, and is thus represented as approximately equal (≈), to signify P >0.05. 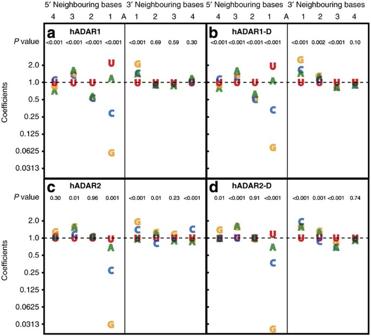Figure 3: Analysis of the coefficients for the eight-term model. The vertical axis of each panel (a–dfor the different ADARs) plots the coefficients used in the eight-term multiplicative regression model (numerical values inSupplementary Data 1). To obtain an estimate of the % editing of a target adenosine, coefficients for each of the eight-base positions are multiplied together, and this value is multiplied by 20 to account for the normalization of the mean % editing to 20% (seeMethods). ThePvalues given for 5′ and 3′ positions (top of each panel) evaluate the null hypothesis that the % editing of the target adenosine is unrelated to the identity of the base at that position; a smallPvalue indicates that at least two of the four possible bases at the indicated position lead to different amounts of editing of the target adenosine. Widely dispersed plot symbols (and lowPvalues) at a particular position indicate a large effect of the identity of the base at that position on the % editing of the target adenosine, whereas overlapping plot symbols (and highPvalues) indicate little or no effect of the identity of the base at that position. Table 3 provides a side-by-side comparison of our refined preferences with those previously published. Although similar, our analyses allow a more quantitative treatment (see Supplementary Data 1 ), and also reveal a previously undetected 3′ neighbour preference for hADAR1. Table 3 Comparison of refined neighbour preferences with those previously determined. Full size table Bases beyond the nearest neighbour affect preferences To test whether editing is influenced by nucleotides beyond the nearest neighbour, we extended the regression analysis to include the second, third and fourth neighbours (see Supplementary Data 1 ). Comparing the R 2 values from left to right in Table 2 , in general, shows better fit as more terms are included for flanking bases. The increased fit when terms are included for the four neighbouring bases on both sides strengthens the observation that ADAR editing is influenced by more than nearest neighbours ( Table 2 , Model #6). The algorithm for this eight-term 1st–4th 5′ and 1st–4th 3′ neighbour fit model is: with coefficients given in Supplementary Data 1 and visually displayed in Figure 3 . To uniquely define coefficient values, all U coefficients with the exception of the first 5′ position were constrained to equal 1. Interestingly, the coefficients for the second 5′ neighbouring base vary substantially from 1 for hADAR1 and hADAR1-D, but not for hADAR2 and hADAR2-D. This suggests that the hADAR1 catalytic domain has structural features that are more interactive with the first and second 5′ nearest neighbours than the hADAR2 catalytic domain. Figure 3: Analysis of the coefficients for the eight-term model. The vertical axis of each panel ( a – d for the different ADARs) plots the coefficients used in the eight-term multiplicative regression model (numerical values in Supplementary Data 1 ). To obtain an estimate of the % editing of a target adenosine, coefficients for each of the eight-base positions are multiplied together, and this value is multiplied by 20 to account for the normalization of the mean % editing to 20% (see Methods ). The P values given for 5′ and 3′ positions (top of each panel) evaluate the null hypothesis that the % editing of the target adenosine is unrelated to the identity of the base at that position; a small P value indicates that at least two of the four possible bases at the indicated position lead to different amounts of editing of the target adenosine. Widely dispersed plot symbols (and low P values) at a particular position indicate a large effect of the identity of the base at that position on the % editing of the target adenosine, whereas overlapping plot symbols (and high P values) indicate little or no effect of the identity of the base at that position. Full size image The P values at the top of each panel in the figure evaluate the null hypothesis that the coefficients of all four bases in the indicated position were identically equal to 1, corresponding to no influence of the bases at that position. The P values reveal a difference between hADAR1 and hADAR2. For hADAR1 and hADAR1-D, the only bases that modelled poorly ( P >0.001) are on the 3′-side of the editing site, after the immediate 3′ neighbour. However, for hADAR2 and hADAR2-D, bases that modelled poorly are on both 5′ and 3′ sides, again excluding the nearest neighbour. This indicates that hADAR1 is not only more sensitive to the second 5′ base identity than hADAR2, but those beyond the second 5′ neighbour. Evaluating the algorithm on perfectly paired dsRNA The eight-term algorithms were tested for their ability to predict editing reported for hADAR1 in 36 and 48 bp dsRNAs, and hADAR2 in 61 and 102 bp dsRNAs [18] ( Fig. 4 ; see Supplementary Fig. S1 ). In the previous report, editing sites were ranked as major (I), minor (i), or below-detection/unedited (A). Using a best fit to experimental data, we defined a boundary for scoring edited (I+i), and unedited (A) sites for hADAR1 (9.6%) and hADAR2 (21%) and found that the eight-term regression algorithms successfully ranked most editing sites above most below-detection/unedited sites ( Fig. 4a ). The hADAR1 algorithm successfully scored sites for 27 of 37 adenosines (73%) and that for hADAR2, 49 of 76 adenosines (64%), reiterating the accuracy of regression analyses ( Table 2 , model #6, hADAR1=77.1%, hADAR2=57.0%). 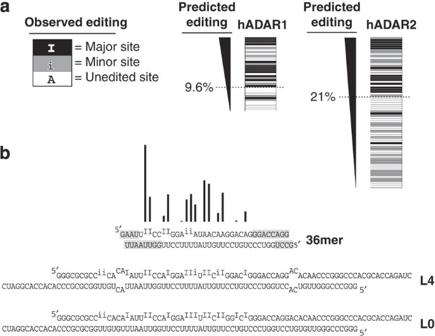Figure 4: The hADAR1 and hADAR2 eight-term nearest neighbour regression models as predictive tools. (a) The major (black), minor (grey) and below-detection/no editing (white) sites of dsRNAs previously reported18are ranked according to percentage of editing predicted by the eight-term best-fit model. In the previously published analysis, the boundary for scoring a site as edited/unedited was dictated by the sensitivity of methods available at the time. We used a best-fit analysis to define this cutoff as 9.6% for hADAR1, and 21% for hADAR2. Locations of editing sites within these dsRNAs are shown inSupplementary Figure S1. (b) Bar height shows relative levels of editing in the 36-bp sequence, as predicted by the eight-term model for hADAR1. The 36-bp dsRNA is shown below as a free molecule, or bounded by internal loops (L4) or additional contiguous base pairs (L0). Published patterns of editing in the three dsRNAs were determined withXenopus laevisADAR1, whose neighbour preferences are identical to those of hADAR1 (ref.18). Editing in the three dsRNAs was determined by primer extension20, with sites qualitatively categorized as major (I) or minor (i). Grey highlighted ends of duplexes represent regions where ADARs are unable to edit due to proximity to termini18. Figure 4: The hADAR1 and hADAR2 eight-term nearest neighbour regression models as predictive tools. ( a ) The major (black), minor (grey) and below-detection/no editing (white) sites of dsRNAs previously reported [18] are ranked according to percentage of editing predicted by the eight-term best-fit model. In the previously published analysis, the boundary for scoring a site as edited/unedited was dictated by the sensitivity of methods available at the time. We used a best-fit analysis to define this cutoff as 9.6% for hADAR1, and 21% for hADAR2. Locations of editing sites within these dsRNAs are shown in Supplementary Figure S1 . ( b ) Bar height shows relative levels of editing in the 36-bp sequence, as predicted by the eight-term model for hADAR1. The 36-bp dsRNA is shown below as a free molecule, or bounded by internal loops (L4) or additional contiguous base pairs (L0). Published patterns of editing in the three dsRNAs were determined with Xenopus laevis ADAR1, whose neighbour preferences are identical to those of hADAR1 (ref. 18 ). Editing in the three dsRNAs was determined by primer extension [20] , with sites qualitatively categorized as major (I) or minor (i). Grey highlighted ends of duplexes represent regions where ADARs are unable to edit due to proximity to termini [18] . Full size image Because the 795-bp dsRNA is long and perfectly base-paired, effects of termini proximity [17] and selectivity [19] are minimal. Thus, our algorithms reflect neighbour preferences largely free of other contributions. This is emphasized by comparing editing sites predicted by the algorithm with experimentally determined editing sites in substrates in which selectivity has variable roles ( Fig. 4b ). A previous study compared ADAR1 editing in a short double-stranded sequence to editing of the same sequence embedded within a larger dsRNA, either bounded by internal loops or contiguous base pairs. Because of effects of selectivity, only a subset of the predicted sites are edited in the short dsRNA, but almost all predicted sites are edited in the context of a longer molecule. Subtle differences may relate to differences in reaction conditions as duplexes in Figure 4b were edited to completion and mapped using primer extension [20] , which only provides semi-quantitative data. Roles of dsRBMs and RNA structure in a natural substrate We also analysed in vitro editing of an RNA mimicking the human 5-HT 2C pre-mRNA, which contains the 'A'–'E' editing sites observed in vivo ( Fig. 5 ). The human 5-HT 2C RNA was incubated with each ADAR, and at the highest concentrations tested (see Methods ), was edited to a similar overall level by hADAR1 (6.3%), hADAR1-D (6.4%), hADAR2 (6.7%) and hADAR2-D (6.6%); editing patterns were independent of protein concentration. 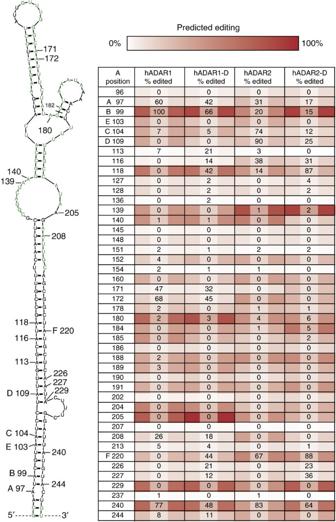Figure 5: Analysis of an endogenous substrate reveals contributions of dsRBMs and RNA structure. A predicted secondary structure in human 5-HT2Cpre-mRNA is illustrated with the 'A'–'E' endogenous editing sites labelled. Sites are numbered from the 5′ G of thein vitrotranscript (seeSupplementary Methodsfor sequence). The 5-HT2Cexon 5/intron 5 boundary is between positions 181/182 (black line). The lowest free-energy structure shown was predicted with Mfold43,44; nucleotides predicted to have alternative pairing within 2 kcal mol−1of the most stable pairing are green. The table shows % of population edited by different ADARs at each measurable adenosine in the illustrated structure; values are normalized to that of hADAR1 to allow comparison. Colour coding shows % editing as predicted from the eight-term model derived from data of the perfectly duplexed 795-bp dsRNA. White represents 0% predicted editing with colour gradations up to dark red (100% predicted editing). These concentrations were chosen for comparison, and % editing values are reported in Figure 5 . Adenosines are numbered to correspond with positions in the secondary structure, and tabulated sites are shaded to indicate likelihood of editing as predicted by our eight-term model. Figure 5: Analysis of an endogenous substrate reveals contributions of dsRBMs and RNA structure. A predicted secondary structure in human 5-HT 2C pre-mRNA is illustrated with the 'A'–'E' endogenous editing sites labelled. Sites are numbered from the 5′ G of the in vitro transcript (see Supplementary Methods for sequence). The 5-HT 2C exon 5/intron 5 boundary is between positions 181/182 (black line). The lowest free-energy structure shown was predicted with Mfold [43] , [44] ; nucleotides predicted to have alternative pairing within 2 kcal mol −1 of the most stable pairing are green. The table shows % of population edited by different ADARs at each measurable adenosine in the illustrated structure; values are normalized to that of hADAR1 to allow comparison. Colour coding shows % editing as predicted from the eight-term model derived from data of the perfectly duplexed 795-bp dsRNA. White represents 0% predicted editing with colour gradations up to dark red (100% predicted editing). Full size image Editing at sites previously observed in vivo recapitulated well in vitro , consistent with studies showing that editing specificity derives from ADAR without a requirement for accessory proteins [26] . As observed in vivo , sites 'A' and 'B' were predominantly edited by hADAR1 (ref. 27 ), and sites 'C' and 'D' were predominantly edited by hADAR2 (refs 27 , 28 ). The specificities of the full-length proteins for these sites were mimicked by their deaminase domains, but the important role of the dsRBMs was apparent in the analysis of the imperfectly paired 5-HT 2C RNA. For example, absence of the dsRBMs correlated with a dramatic loss of efficiency in editing at sites 'C' and 'D' by hADAR2. Analyses of endogenous RNA indicate that site 'E' is a poorly edited site [29] , and we did not observe in vitro editing at site 'E' with any ADAR. Intronic site 'F' is also edited in vivo , although its significance and which ADAR(s) edit this site are unclear [30] . We observed editing at site 'F' with all proteins except full-length hADAR1, implying ADAR1's dsRBMs sometimes block editing. Although the shading of the 'A'–'E' sites ( Fig. 5 ) reveals that our eight-term model predicted editing at these sites, it performed poorly in predicting the relative amount of editing with different ADARs, again suggesting that non-canonical features that disrupt a base-paired dsRNA have a key role in editing specificity. Further, at most sites the tint of the shading was similar for the full-length ADAR and its catalytic domain, consistent with our observation that dsRBMs do not significantly change the sequence preferences observed with a completely base-paired dsRNA ( Fig. 2a,b ). In contrast, for many editing sites the percent in vitro editing observed in the 5HT 2C RNA substrate was dramatically affected by the presence of the dsRBMs. This suggests that dsRBMs have a larger role in RNA containing mismatches, bulges and loops, such as the 5HT 2C RNA. Other sites predicted as editing 'hot-spots' by our model, but not edited, or poorly edited, in vitro , were mostly within unpaired regions, or near the boundary of a predicted stem and an unpaired region (139, 140, 180, 205, 229); this is consistent with the fact that ADARs preferentially edit highly base-paired sequences. We also observed in vitro editing at sites in addition to those reported as being edited in vivo . Many of these were predicted by our model to be edited, albeit in most cases the relative amount of editing predicted for the four ADARs differed from that observed in vitro (for example, see positions 116, 118, 171, 172, 208, 240, 244). In most cases, differences were best understood by considering that structural disruptions in the 5HT 2C RNA substrate uncouple helices to approximate a series of short double-stranded regions [20] . Several additional conclusions emerged. First, adenosines at positions 171, 172 and 208 were edited in vitro to varying degrees by hADAR1 and hADAR1-D, but not by hADAR2 and hADAR2-D, even though our model predicted greater editing by hADAR2. This indicates that hADAR1 and hADAR2 are affected differently by RNA structure. Further, at these same positions, preferences of the full-length proteins tracked with those of their deaminase domains, implying that the catalytic domain alone can discriminate structural features. Finally, certain positions were edited by the catalytic domain but not by the full-length ADAR (for example, 226, 227), even at sites predicted to be in preferred contexts. Thus, for both ADARs, dsRBMs may sometimes block editing sites. Similarly, adenosines at positions 116 and 118, like site 'F', are edited by all proteins except full-length hADAR1, implying these sites are blocked by dsRBMs of hADAR1, but not those of hADAR2. We show that current protocols for Sanger sequencing allow ADAR editing to be quantified from peak heights of cDNA sequence traces with a decreased error than previous methods (s.d. ≤5%; Table 1 ). Using this methodology, we refined and quantified neighbour preferences for human ADAR1 and ADAR2. In addition, we applied our methodology to answer questions about ADARs and to generate an algorithm for the de novo prediction of editing sites in dsRNA. Differences between preferences detailed here and those previously reported ( Table 3 ) [17] , [18] are explained by an increased accuracy and larger sample size, and the different in vitro conditions used. Previous studies used data from dsRNA reacted to completion, thus sacrificing the ability to detect differences between well-edited sites. To overcome this limitation, we reacted 795-bp dsRNA to an intermediate level of editing. Previous studies used dsRNA that was very short compared with the 795-bp dsRNA, incurring effects of duplex termini [17] , [18] , and selectivity [19] . We consider data from the 795-bp dsRNA to reflect neighbour preferences largely free of these effects. Even with their limitations, previous studies reported neighbour preferences that agree fairly closely with those reported here ( Table 3 ). However, our refinement allowed discrimination between nearest neighbours that were previously thought to be targeted equally well, and also revealed a 3′ nearest neighbour preference for hADAR1. Further, our larger data sets allowed us to construct regression models that allow new insight into ADAR preferences (below). A prevailing hypothesis is that dsRBMs anchor an ADAR to a dsRNA region, while the catalytic domain provides the specificity that leads to a preference for certain adenosines [21] . Indeed, chimeric proteins of human ADAR1 and ADAR2, in which the catalytic domains are exchanged, show specificity that tracks with catalytic domain identity [31] . By carefully comparing preferences of full-length hADAR1 and hADAR2 with those of their catalytic domains, we confirm that, for most triplet contexts, this hypothesis is true. However, our more quantitative approach allowed us to discern that full-length hADAR2, compared with its catalytic domain, has an increased preference for adenosines with a 3′ G ( Figs 2b and 3 ). Thus, we find that dsRBMs of hADAR2 contribute to editing specificity. This agrees with nuclear magnetic resonance solution data indicating that serine 258 in the second dsRBM of rat ADAR2 forms a hydrogen bond with the minor groove amino group of the guanosine 3′ to the R/G editing site [15] . We note, however, that our analyses indicate the catalytic domain, not the dsRBMs, is largely responsible for discriminating adenosines in different sequence contexts. We found that a multiplicative model that separately considers the identity of 5′ and 3′ nearest neighbours gives as good a fit to editing data as triplet identities. This suggests that the ADAR active site interrogates these positions independently. Further, multiplicative models that considered base identities beyond nearest neighbours showed increased fit ( Table 2 ), indicating that editing site choice is influenced by more than nearest neighbours. Finally, the regression modelling indicated that, for all proteins studied, 5′ bases have more influence on editing than 3′ bases. Our analysis revealed that hADAR1 is more influenced by bases 5′ of an editing site than hADAR2 ( Fig. 3 , P values). At the surface of the hADAR2 catalytic pocket are amino acids that are disordered in the crystal structure [14] , and show poor conservation with hADAR1. The hADAR1a sequence (GALFDKSCSDRAMESTESRHYPVFENPKQGK) is also slightly longer than the analogous hADAR2a sequence (ARIFSPHEPILEEPADRHPNRKARGQ). In the hADAR2-D crystal structure, this region is predicted to be close to the site being edited, and thus, is a good candidate for mediating the increased sensitivity of hADAR1 to 5′ neighbours. We developed a web-based application based on our eight-term model ( http://www.biochem.utah.edu/bass/inosinepredict ; Supplementary Software ). The algorithm was developed by fitting to experimentally determined editing sites in a long perfectly base-paired dsRNA, and approximates ADAR preferences in the absence of the effects of RNA structure. ADARs target dsRNA formed from sense–antisense transcripts [32] , or that introduced into an organism to mediate RNA interference [33] , and we envision our algorithm facilitating researchers in the identification of such sites. That said, although our algorithm represents an advance, the R 2 values ( Table 2 ) emphasize that its predictive power is still limited. Predictions should be treated cautiously, especially for hADAR2, or for approximating editing under conditions different from those used here. However, we envision the limitations of our model are key to its improvement. For example, application of our algorithm to ADAR substrates in which RNA structure mediates editing site choice will facilitate studies to define how structure affects editing, setting the stage for future algorithms that take such features into account. Protein purification Expression constructs included an N-terminal 10-histidine tag followed by a TEV protease site, then the ADAR cDNA, ligated into the YEpTOP2PGAL1 vector [34] . hADAR2 and hADAR2-D vectors were constructed as described using a hADAR2a cDNA template [35] , [36] , with the hADAR2-D construct encoding residues 299–701 of hADAR2a [14] . hADAR1 and hADAR1-D vectors were similarly constructed from the nuclear hADAR1a isoform, which initiates at Met296 of the hADAR1d isoform [37] . The hADAR1-D construct encodes residues 528–931 of hADAR1a. Proteins were expressed in Saccharomyces cerevisiae and purified as described [36] , with modifications specified in Supplementary Methods . hADAR2, hADAR2-D and hADAR1-D were purified to >98% as estimated by SYPRO Red staining of SDS–polyacrylamide gels with BSA standards [18] , and stored in storage buffer A (20 mM Tris–HCl, pH 8.0, 100 mM NaCl, 1 mM 2-mercaptoethanol, 15% glycerol). hADAR1 was stored in storage buffer B (50 mM Tris–HCl, pH 8.0, 200 mM KCl, 5 mM EDTA, 0.01% NP-40, 10% glycerol and 1 mM DTT [35] ) and purified to 80%, twice the purity previously achieved for hADAR1 (ref. 18 ). RNA preparation Radiolabelled and non-radiollabeled 795-bp dsRNA encoding chloramphenicol acetyl transferase (CAT) was prepared as described [38] . The dsRNA has 22 nt 5′ overhangs at each termini. Human 5-HT 2C pre-mRNA template was cloned de novo with a T7 RNA polymerase promoter into the pUC18 vector (Fermentas; all primers in Supplementary Table S2 ). Transcription was as for 795-bp dsRNA [38] . RNA (sequence in Supplementary Methods ) was gel purified, boiled (2 min) and refolded as for hybridization of 795-bp dsRNA [38] ; editing was identical without gel purification or refolding. Four-dye-trace bulk sequencing quantification cDNA populations from reverse transcription PCR (RT–PCR) of editing products were bulk sequenced in one reaction rather than sequencing individually cloned molecules. Thus, editing sites appear as mixed peaks in traces. Four-dye-trace sequences in abi file format were processed using BioEdit ( http://www.mbio.ncsu.edu/BioEdit/bioedit.html ; File>Batch Export of Raw Sequence Trace Data). Text file outputs were opened and evaluated in Microsoft Excel (Microsoft). Editing sites were quantified by measuring maximal height of T peaks (unedited) and C peaks (edited) and calculating percentage of the population edited at each site (100%×[C height/(T height+C height)]). For peaks without a clear maximal height, shoulder shape and distances between distinct peaks were used as guides to manually select a shoulder value as the maximal peak height. For method validation, standard techniques were used to clone a transcription template that differed from the antisense CAT template [38] in that certain adenosines were changed to guanosines ('edited'). Primer pair 31/32, flanking the CAT coding region, was used to PCR amplify edited and unedited CAT antisense templates. PCR products were gel purified and concentrations determined by ultraviolet spectroscopy, using precise extinction coefficients, calculated as described [39] . PCR products were mixed in known ratios to mimic prescribed levels of editing at certain adenosines, then sequenced (Primer 55; GENEWIZ). ADAR assays For ADAR activity assays, radiolabelled 795-bp dsRNA was reacted in 22 mM Tris–HCl, pH 7.5 (25 °C), 40 mM KCl, 10 mM NaCl, 6.5% glycerol, 0.5 mM DTT, 0.1 mM 2-mercaptoethanol, 0.01% NP-40 and 1 U μl −1 Promega RNasin Plus (Promega), for 1 h at 30 °C. Varying concentrations (nM–μM) of hADAR2 and hADAR2-D were incubated with 1 nM 795-bp dsRNA, and hADAR1 and hADAR1-D with 0.1 nM 795-bp dsRNA, to determine conditions that provided ∼ 20% overall A-to-I conversion, as determined by thin layer chromatography [40] . For the ADAR preference assay, non-radiolabelled 795-bp dsRNA was reacted as in the ADAR activity assay. ADAR concentrations were chosen to give ∼ 20% A-to-I conversion in 1 h (hADAR1, 2 nM; hADAR1-D, 80 nM; hADAR2, 2 nM; hADAR2-D, 400 nM). Reactions were stopped by vortexing with phenol and purified [14] . Edited RNA product was reverse transcribed (Thermoscript, Invitrogen; primer 51, antisense strand; primer 52 sense strand), treated with RNAse H, and single-stranded DNA PCR amplified with Platinum Pfx DNA Polymerase (Invitrogen). Primer pair 52/54 was used to amplify sense strand, and primer pair 51/53 antisense strand. RT–PCR products were gel purified or purified with ExoSAP-IT (USB) before sequencing. Sequencing primers were 52, 56, 58, 64, 66 and 68 (sense strand) and 51, 55, 57, 63, 65, 67, 69 and 73 (antisense strand). Primer extension sequencing was by GENEWIZ using Applied Biosystems BigDye version 3.1 and run on Applied Biosystem's 3730xl DNA Analyzer (Applied Biosystems). 5HT 2C pre-mRNA was incubated (30 °C, 4 h) with increasing ADAR concentration, while the RNA concentration was kept at 0.1 nM; hADAR1 0.5, 2, 10 and 187 nM; hADAR1-D 20, 80 400 and 675 nM; hADAR2 0.5, 2, 10 and 17.4 nM; hADAR2-D 100, 400, 800 and 1,938 nM. Reactions were stopped with Proteinase K (NEB) and SDS and purified [41] . Primer 90 was used for reverse transcription of 5HT 2c RNA, and primer pair 91/92 for PCR. The purified RT–PCR product was sequenced (primer 76, GENEWIZ), and editing calculated from traces as for 795-bp dsRNA. Statistical methods Unadjusted % editing values at a given site were normalized before statistical analyses to eliminate systematic experimental deviations between results obtained for the four ADARs. For each enzyme, denoted by the index i , i =1, 2, 3 or 4, normalized % editing values were computed as: normalized % editing=A[i]+B[i]×[unadjusted % editing], where the coefficients A[i] and B[i] were computed using equations derived from the following constraints: (1) the mean % editing across all 406 occurrences of the base 'A' in the 795-bp dsRNA was set to 20%, and (2) for each of the four enzymes, the mean % editing when the 5′ base was 'G' was set to the overall average % editing. These normalizations allowed comparison between preferences of different enzymes even though the overall average editing ranged from 16.4 to 22.7%. After normalization, a series of regression models were fit for each enzyme to summarize the dependence of editing on the configuration of neighbouring bases. The regression models related the normalized % editing results for each adenosine to the following factors: Model 1: The 16 combinations of the four 5′ and the four 3′ bases (triplet model) Model 2: The immediate 5′ base only Model 3: Both the immediate 5′ and immediate 3′ bases assuming a multiplicative relationship: normalized % editing=[B1 if 5′ base=A, B2 if 5′ base=C, B3 if 5′ base=G, B4 if 5′ base=U]×[1 if 3′ base=U, A1 if 3′ base=A, A2 if 3′ base=C, and A3 if 3′ base=G], Model 4: Extension of model 3 to account for both the 1st and 2nd 5′ bases and the 1st and 2nd 3′ bases. Model 5: Extension of model 3 to account for the 1st, 2nd and 3rd 5′ bases and the 1st, 2nd and 3rd 3′ bases. Model 6: Extension of model 3 to account for the 1st, 2nd, 3rd and 4th 5′ bases and the 1st, 2nd, 3rd and 4th 3′ bases. A multiplicative structure for Models 3, 4, 5 and 6 was used because these models fit the data substantially better than additive models. The coefficients of each model were estimated using either linear (models 1 and 2) or nonlinear (models 3, 4, 5, and 6) least squares regression. The explanatory power of the models was quantified by adjusted R 2 values [42] , which indicate percent of the variance in the normalized % editing results across the 406 adenosines, which could be explained by each model, with an adjustment for the degrees of freedom of each model. A bootstrap resampling procedure using 2,000 independent bootstrap samples was developed to perform statistical inferences to account for the initial normalization and large differences in variance of % editing values between different neighbouring base configurations. The normalization step was repeated with each bootstrap sample, and to account for the differences in variances, resampling was stratified by the combination of the immediate 5′ and 3′ bases. The bootstrap results were used to compute standard errors for quantities of interest. P values and 99% confidence intervals were then computed based on normal approximations. Because many comparisons were performed, differences in preferences were regarded as statistically significant if the two-sided P value <0.01. No further multiple comparison adjustment was performed. Under our bootstrap approach, P values and confidence intervals were determined based on variation in % editing results across the 406 A-bases over the length of the RNA. This contrasts with the alternative approach of performing statistical inferences based on variation between experimental replications. How to cite this article: Eggington, J. M. et al . Predicting sites of ADAR editing in double-stranded RNA. Nat. Commun. 2:319 doi: 10.1038/ncomms1324 (2011).